Direct neuronal glucose uptake heralds activity-dependent increases in cerebral metabolism Metabolically, the brain is a highly active organ that relies almost exclusively on glucose as its energy source. According to the astrocyte-to-neuron lactate shuttle hypothesis, glucose is taken up by astrocytes and converted to lactate, which is then oxidized by neurons. Here we show, using two-photon imaging of a near-infrared 2-deoxyglucose analogue (2DG-IR), that glucose is taken up preferentially by neurons in awake behaving mice. Anaesthesia suppressed neuronal 2DG-IR uptake and sensory stimulation was associated with a sharp increase in neuronal, but not astrocytic, 2DG-IR uptake. Moreover, hexokinase, which catalyses the first enzymatic steps in glycolysis, was highly enriched in neurons compared with astrocytes, in mouse as well as in human cortex. These observations suggest that brain activity and neuronal glucose metabolism are directly linked, and identiy the neuron as the principal locus of glucose uptake as visualized by functional brain imaging. Functional brain imaging has, in recent years, revolutionized our understanding of complex neural processing. Positron emission tomography (PET) imaging of glucose analogues takes advantage of the fact that glucose is the major energy substrate that fuels neural activity. Unlike other organs, the brain does not use fatty acid oxidation as a source of energy and is highly dependent on glucose for sustenance [1] , [2] . However, a point of contention is that functional imaging techniques rely on surrogate markers of neural activity and thus leave questions as to whether a direct relationship exists between neuronal activity and metabolic surrogates. Interpretation of activity-dependent glucose uptake is complex due to competing theories of central nervous system (CNS) glucose metabolism. According to one theory, the astrocyte-to-neuron lactate shuttle hypothesis, energy metabolism is compartmentalized and glycolysis is outsourced to astrocytes [3] , [4] , [5] , [6] , [7] , [8] . This model proposes that glucose is primarily taken up by astrocytes located around blood vessels and converted to lactate. In turn, neuronal energy metabolism relies chiefly on import of lactate and the energetically favourable process of mitochondrial lactate oxidation [3] , [4] , [5] , [6] , [7] . A consequence of the astrocyte-to-neuron lactate shuttle hypothesis is that glucose metabolism in activated brain regions only indirectly reflects neuronal metabolism, and that functional brain imaging might not provide accurate information concerning neuronal activity. The opposing view is the parsimonious hypothesis that neurons take up glucose directly from the interstitium and generate ATP from both glycolysis and oxidative metabolism [9] , [10] , [11] , [12] . To correctly interpret human brain imaging, it is therefore of defining importance to discern which population of cells increases glucose uptake during complex neural processing. Here we have used in vivo two-photon imaging of a near-infrared glucose analogue to assess cellular glucose uptake [13] , [14] . We report findings that support the parsimonious model by showing that neurons, and not astrocytes, during rest as well as during activity-dependent increases in neural activity, are the primary consumers of glucose. Further experiments used a combination of genomic expression analysis and quantitative immunohistochemistry to evaluate neuronal versus astrocytic expression of hexokinases (HKs). HKs catalyse the first step of glycolysis in which glucose is converted to glucose-6-phosphate. All the intermediary products of the glycolytic pathway, including glucose-6-phosphate, are impermeable to the plasma membrane and are, thereby, trapped within the cytosol. Products of glycolysis can first exit the cells after they are metabolized to either pyruvate or lactate, or oxidized to CO 2 and H 2 O (refs 15 , 16 ). Accordingly, HK can be regarded as the gatekeeper enzymatic step of glycolysis, as their expression correlates directly with the rate of glucose metabolism across multiple regions, including the cortex, hippocampus and retina [17] . Our analysis showed that neurons consistently expressed higher levels of HKs than astrocytes in both mouse and human brain. Validation of the 2DG-IR glucose probe A major challenge in assessing neuronal and astrocyte energy metabolism has been the inability to image glucose uptake with cellular resolution in vivo. The majority of studies on neuronal versus astrocytic glucose uptake have therefore been limited to cell culture or brain slice models. In the pursuit of improving the analysis of cellular glucose uptake, we assessed a near-infrared 2-deoxyglucose probe (IRDye 800CW 2DG, 2DG-IR). Owing to its low energy wavelength absorption, this compound is used for imaging of glucose consumption in live animals and can reliably track tumour growth in vivo [13] , [14] . We first compared 2DG-IR uptake with that of 14 C-glucose and 14 C-2-deoxyglucose ( 14 C-2DG) in both primary neurons and astrocytes in vitro [18] , [19] ( Fig. 1a ). The initial analysis showed that cultured neurons exhibited a fourfold higher rate of glucose uptake ( 14 C-glucose) than cultured astrocytes ( Fig. 1b ). The glucose analogue, 14 C-2DG, was also taken up several fold faster in neuronal than astrocytic cultures ( Fig. 1c ). Radiolabelled 2DG has been extensively used to study functional activation, as Sokoloff and colleagues [20] discovered that 2DG after its phosphorylation to glucose-6-phosphate is trapped in neural cells due to the low expression of glucose-6 phosphatase in the brain. In particular, [ 18 F]2-fluoro-2-deoxy-D-glucose ( 18 FDG) has routinely been employed in PET studies to identify activity-dependent increases in local metabolic activity in human subjects [21] . To obtain cellular resolution of glucose uptake, we next compared the uptake of the near-infrared 2DG glucose analogue (2DG-IR) in cultured neurons and astrocytes to that of 14 C-2DG. Similar to 14 C-2DG uptake, neurons exhibited a several fold higher rate of 2DG-IR uptake than astrocytes ( Fig. 1c ). Substrate competition analysis showed that D -glucose suppressed 14 C-2DG and 2DG-IR uptake in a concentration-dependent manner ( Fig. 1d ). Moreover, cytochalasin B, a nonspecific glucose transport inhibitor, also strongly inhibited the uptake of 14 C-glucose, 14 C-2DG and 2DG-IR in neuronal and astrocytic cultures ( Fig. 1e,f ). 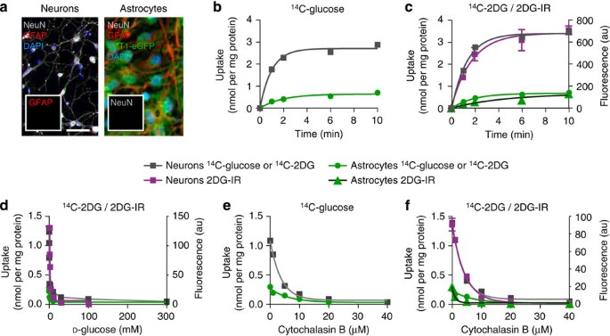Figure 1: Preferential neuronal uptake of glucose and glucose analoguesin vitro. (a) Immunocytochemistry of NeuN (grey), GFAP (red) and DAPI (blue) in neuronal cultures from wild-type mice (left) and astrocyte cultures from GLT1-eGFP mice (right). Insert: GFAP (left) and NeuN (right) staining signals alone showed no staining signals. Scale bar, 50 μm. (b)14C-glucose uptake, and (c)14C-2DG and 2DG-IR uptake in neurons and astrocytes plotted as a function of time. Slopes for initial linear phase14C-glucose neurons, 1.15±0.06;14C-glucose astrocytes, 0.20±0.01;14C-2DG neurons, 1.39±0.03;14C-2DG astrocytes, 0.23 ±0.01 (nmol per mg protein min−1); 2DG-IR neurons, 245.00±30.52; 2DG-IR astrocytes, 28.17±1.41 (in arbitrary units, au min−1). (d) Substrate competition of14C-2DG and 2DG-IR uptake plotted as a function of increasing concentration ofD-glucose (Ki in mM:14C-2DG neurons, 0.41±0.01; 2DG-IR neurons, 0.87±0.04;14C-2DG astrocytes, 0.71±0.0). (e) Effect of increasing concentrations of the nonspecific glucose transporter inhibitor, cytochalasin B, on14C-glucose uptake (Ki in μM:14C-glucose neurons, 2.58±0.11;14C-glucose astrocytes, 4.39±0.03). (f) The effect of cytochalasin B effect on14C-2DG and 2DG-IR uptake (Ki in μM:14C-2DG neurons, 2.59±0.04; 2DG-IR neurons, 3.02±0.23;14C-2DG astrocytes, 4.64±0.06; 2DG-IR astrocytes, 1.66±0.06). The cultures were pretreated with cytochalasin B for 10 min before addition of14C-glucose,14C-2DG, or 2DG-IR. All values are expressed as mean±s.e.m. Figure 1: Preferential neuronal uptake of glucose and glucose analogues in vitro . ( a ) Immunocytochemistry of NeuN (grey), GFAP (red) and DAPI (blue) in neuronal cultures from wild-type mice (left) and astrocyte cultures from GLT1-eGFP mice (right). Insert: GFAP (left) and NeuN (right) staining signals alone showed no staining signals. Scale bar, 50 μm. ( b ) 14 C-glucose uptake, and ( c ) 14 C-2DG and 2DG-IR uptake in neurons and astrocytes plotted as a function of time. Slopes for initial linear phase 14 C-glucose neurons, 1.15±0.06; 14 C-glucose astrocytes, 0.20±0.01; 14 C-2DG neurons, 1.39±0.03; 14 C-2DG astrocytes, 0.23 ±0.01 (nmol per mg protein min −1 ); 2DG-IR neurons, 245.00±30.52; 2DG-IR astrocytes, 28.17±1.41 (in arbitrary units, au min −1 ). ( d ) Substrate competition of 14 C-2DG and 2DG-IR uptake plotted as a function of increasing concentration of D -glucose (Ki in mM: 14 C-2DG neurons, 0.41±0.01; 2DG-IR neurons, 0.87±0.04; 14 C-2DG astrocytes, 0.71±0.0). ( e ) Effect of increasing concentrations of the nonspecific glucose transporter inhibitor, cytochalasin B, on 14 C-glucose uptake (Ki in μM: 14 C-glucose neurons, 2.58±0.11; 14 C-glucose astrocytes, 4.39±0.03). ( f ) The effect of cytochalasin B effect on 14 C-2DG and 2DG-IR uptake (Ki in μM: 14 C-2DG neurons, 2.59±0.04; 2DG-IR neurons, 3.02±0.23; 14 C-2DG astrocytes, 4.64±0.06; 2DG-IR astrocytes, 1.66±0.06). The cultures were pretreated with cytochalasin B for 10 min before addition of 14 C-glucose, 14 C-2DG, or 2DG-IR. All values are expressed as mean±s.e.m. Full size image Collectively, our in vitro analysis showed that neurons outcompete astrocytes with regard to uptake of glucose itself, as well as with uptake of radio- and fluorescence-labelled 2DG. Moreover, the similarities of response to substrate inhibition and cytochalasin B inhibition suggest that both 14 C-2DG and 2DG-IR uptake is dependent on plasma membrane glucose transporters, as previously documented for 14 C-2DG and another fluorescent 2DG analogue, 2-NBDG [22] , [23] . In vivo two-photon imaging of 2DG-IR in awake mice To compare neuronal versus astrocytic 2DG-IR uptake in vivo , we next administered 2DG-IR into the peri-arterial Virchow–Robin space surrounding large penetrating cortical arteries. Using in vivo two-photon excitation, the influx of 2DG-IR along the peri-arterial and peri-capillary space was visualized in astrocyte reporter mice (GLT1-eGFP). Cerebrospinal fluid (CSF) influx of glucose along the peri-vascular space mimics the delivery of glucose that cross the blood–brain barrier (BBB): glucose delivered by the vasculature or by CSF must in both cases pass the peri-vascular space before gaining access to neurons and astrocytes ( Fig. 2a ). Indeed, 2DG-IR was rapidly transported down along the peri-arterial and peri-capillary space. Real-time imaging showed that 2DG-IR moved quickly along the Virchow–Robin space and dispersed from the capillaries evenly into the parenchyma ( Fig. 2b,c ). We then assessed cellular 2DG-IR uptake in reporter mice in vivo ( Fig. 2d ). Neurons identified in CamK2a-tdTomato reporter mice displayed consistently higher 2DG-IR signal than surrounding neuropil, whereas the 2DG-IR signal in GLT1-eGFP + astrocytes was either lower than or did not differ from the surroundings ( Fig. 2d ). However, the high background signal of the untrapped 2DG-IR probe did not permit quantitative analysis of either neuronal or astrocytic 2DG-IR uptake. 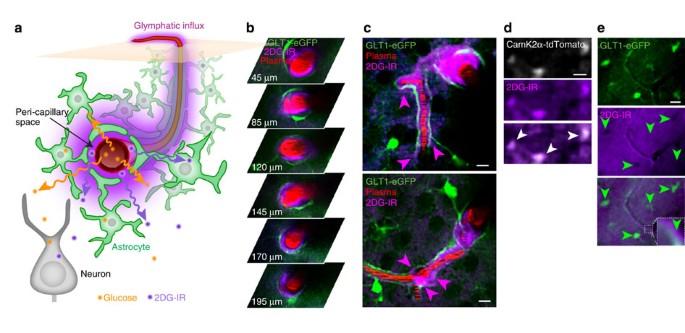Figure 2:In vivoimaging of cellular uptake of a near-infrared glucose analogue, 2DG-IR. (a) Diagram illustrating the entry route of 2DG-IR via the peri-arterial space. 2DG-IR can be delivered either to the CSF via injection in cisterna magna or via micro-injection in the peri-arterial space surrounding cortical penetrating arteries. The CSF influx pathway is similar to vascular delivery of glucose, as glucose must, after crossing the BBB, pass the peri-vascular space before gaining access to neurons and astrocytes. (b) Representative high magnificationin vivoimages at serial depths of 2DG-IR in peri-arterial space surrounding penetrating arteriole at 5 min after injection (N=8). (c) 2DG-IR is transported along the peri-vascular space around both arteries and capillaries followed by diffusion into the tissue 5 min after injection (white arrows) (N=8). (d) 2DG-IR uptake in a CamK2a-tdTomato neuronal reporter mouse showing that the highest 2DG-IR signal co-localizes with CamK2a-tdTomato+neuronal cell bodies (white arrows) (N=3). (e) In contrast, 2DG-IR uptake in GLT1-eGFP+astrocytes (green arrows) is either lower or comparable to surrounding neuropil (N=8). Insert: higher magnification of the capillary wall showing that the high 2DG-IR signal is localized in the peri-capillary space and surrounded by eGFP+vascular endfeet of astrocytes. Scale bars, 10 μm (c,d,e). Figure 2: In vivo imaging of cellular uptake of a near-infrared glucose analogue, 2DG-IR. ( a ) Diagram illustrating the entry route of 2DG-IR via the peri-arterial space. 2DG-IR can be delivered either to the CSF via injection in cisterna magna or via micro-injection in the peri-arterial space surrounding cortical penetrating arteries. The CSF influx pathway is similar to vascular delivery of glucose, as glucose must, after crossing the BBB, pass the peri-vascular space before gaining access to neurons and astrocytes. ( b ) Representative high magnification in vivo images at serial depths of 2DG-IR in peri-arterial space surrounding penetrating arteriole at 5 min after injection ( N =8). ( c ) 2DG-IR is transported along the peri-vascular space around both arteries and capillaries followed by diffusion into the tissue 5 min after injection (white arrows) ( N =8). ( d ) 2DG-IR uptake in a CamK2a-tdTomato neuronal reporter mouse showing that the highest 2DG-IR signal co-localizes with CamK2a-tdTomato + neuronal cell bodies (white arrows) ( N =3). ( e ) In contrast, 2DG-IR uptake in GLT1-eGFP + astrocytes (green arrows) is either lower or comparable to surrounding neuropil ( N =8). Insert: higher magnification of the capillary wall showing that the high 2DG-IR signal is localized in the peri-capillary space and surrounded by eGFP + vascular endfeet of astrocytes. Scale bars, 10 μm ( c , d , e ). Full size image Quantitative analysis shows that 2DG-IR uptake is highest in neurons To obtain quantitative data of in vivo 2DG-IR uptake in neurons and astrocytes, we next developed an approach to image 2DG-IR signal in awake behaving mice with high cellular resolution: 2DG-IR was administered into CSF via injection into the cisterna magna to overcome the low BBB permeability of fluorescently tagged glucose analogues. Cisterna magna injection also allowed analysis of multiple brain regions, as CSF is distributed brainwide by the glymphatic system ( Fig. 3a ). As previously shown, CSF is rapidly pumped in along penetrating arteries and mixes with interstitial fluid by convective transport supported by astrocytic AQP4 channels [24] , [25] . Thirty minutes after CSF administration of 2DG-IR, the mice were perfusion fixed and vibratome sections were prepared immediately. To reduce background signal, the slices were washed to remove untrapped 2DG-IR ( Fig. 3a ). The use of GLT1-eGFP reporter mice in combination with nuclear labelling (yellow-Hoechst) enabled a side-by-side comparison of neuronal versus astrocytic 2DG-IR uptake. We took advantage of the observation that the diameter of neuronal nuclei (10.2±0.7 μm) is 43.7% larger than that of astrocytes (7.1±0.1 μm, P =0.01, t -test, N =3 mice) and defined neurons as cells with a round nuclei >9 μm and absence of enhanced green fluorescent protein (eGFP; Fig. 3b ). This ex vivo analysis showed that neurons throughout CNS, including the cortex, striatum and hippocampal layers CA1 and CA3 exhibited on average 2.2-fold higher 2DG-IR uptake than astrocytes in awake mice ( Fig. 3c,d ). In particular, CA1 pyramidal neurons in the hippocampus, which are metabolically highly active, displayed a 2.9-fold higher uptake of 2DG-IR than neighbouring astrocytes. 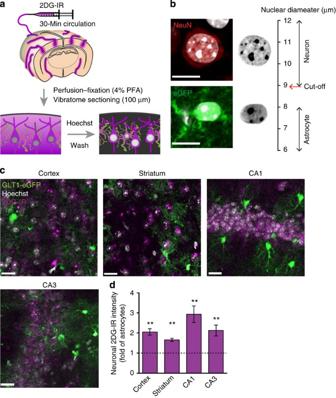Figure 3: Quantitative comparison of neuronal and astrocytic uptake of 2DG-IR. (a) Diagram illustrating entry of 2DG-IR into the brain via peri-arterial routes following CSF injection in GLT1-eGFP reporter mice. After 30 min circulation of 2DG-IR, the animals are perfusion fixed with 4% paraformaldehyde and 100-μm-thick vibratome sections prepared. Before imaging, the slices are washed repeatedly to remove the glucose analogue not trapped in the cytosol and the nuclei were stained with yellow-Hoechst. (b) Neurons were identified in the freshly prepared vibratome sections by their large round nuclei and the absence of cytosolic eGFP (10.2±0.7 μm diameter). Astrocytes were recognized by their smaller nuclei and eGFP signal (7.1±0.1 μm diameter,P=0.01,t-test.N=3 mice). Scale bars, 10 μm. (c) Representative images of 2DG-IR uptake by neurons and astrocytes in the cortex, striatum, CA1 and CA3 in awake GLT1-eGFP mice. Nuclei were stained with yellow-Hoechst (white). Scale bars, 20 μm. (d) Quantification of the ratio of 2DG-IR uptake in neurons versus astrocytes.P<0.001 in the cortex and striatum,P=0.002 in CA1,P=0.006 in CA3, pairedt-test, neurons compared with astrocytes (N=9, 6, 8 and 7 for cortex, striatum, CA1 and CA3, respectively). Bar graphs represent mean±s.e.m. Figure 3: Quantitative comparison of neuronal and astrocytic uptake of 2DG-IR. ( a ) Diagram illustrating entry of 2DG-IR into the brain via peri-arterial routes following CSF injection in GLT1-eGFP reporter mice. After 30 min circulation of 2DG-IR, the animals are perfusion fixed with 4% paraformaldehyde and 100-μm-thick vibratome sections prepared. Before imaging, the slices are washed repeatedly to remove the glucose analogue not trapped in the cytosol and the nuclei were stained with yellow-Hoechst. ( b ) Neurons were identified in the freshly prepared vibratome sections by their large round nuclei and the absence of cytosolic eGFP (10.2±0.7 μm diameter). Astrocytes were recognized by their smaller nuclei and eGFP signal (7.1±0.1 μm diameter, P =0.01, t -test. N =3 mice). Scale bars, 10 μm. ( c ) Representative images of 2DG-IR uptake by neurons and astrocytes in the cortex, striatum, CA1 and CA3 in awake GLT1-eGFP mice. Nuclei were stained with yellow-Hoechst (white). Scale bars, 20 μm. ( d ) Quantification of the ratio of 2DG-IR uptake in neurons versus astrocytes. P <0.001 in the cortex and striatum, P =0.002 in CA1, P =0.006 in CA3, paired t -test, neurons compared with astrocytes ( N =9, 6, 8 and 7 for cortex, striatum, CA1 and CA3, respectively). Bar graphs represent mean±s.e.m. Full size image Anaesthesia predominantly supresses neuronal 2DG-IR uptake We then explored the question of whether anaesthesia differentially suppresses neuronal versus astrocytic energy metabolism. Initial experiments based on the classical quantitative autoradiographic measurements of 14 C-2DG confirmed that ketamine/xylazine anaesthesia potently decreased cortical glucose utilization ( Fig. 4a ) [26] , [27] , [28] . Interestingly, we found that ketamine/xylazine anaesthesia also significantly decreased the ratio of neuronal versus astrocytic 2DG-IR uptake based on analysis of 2DG-IR signal in GLT1-eGFP reporter mice ( Fig. 4b ). Thus, anaesthesia-induced suppression of glucose metabolism predominantly reflects a suppression of neuronal, rather than astrocytic, glucose uptake. 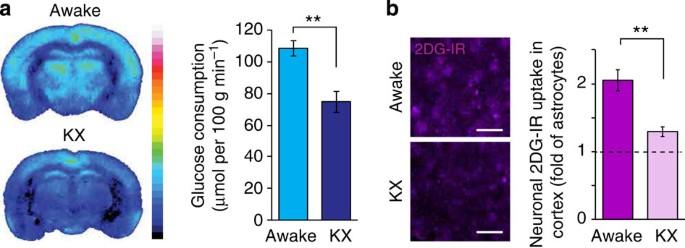Figure 4: Anaesthesia preferentially reduces neuronal 2DG-IR uptake. (a) Left: representative14C-2DG autoradiographs of awake and anaesthetized mice. Right: quantifications of glucose consumption based on14C-2DG autoradiography in the cortex of awake and ketamine/xylazine-anaesthetized mice.P=0.001,t-test (N=5). (b) Left: imaging of 2DG-IR in the cortex of awake and mice anaesthetized with ketamine 100 mg kg−1and xylazine 10 mg kg−1, intraperitoneally (i.p.; KX). Scale bars, 20 μm. Right: anaesthesia reduced the ratio of neuronal versus astrocytic 2DG-IR uptake in the cortex.P=0.002, Mann–Whitney test,N=9 awake,N=6, anaesthetized. Bar graphs represent mean±s.e.m. Figure 4: Anaesthesia preferentially reduces neuronal 2DG-IR uptake. ( a ) Left: representative 14 C-2DG autoradiographs of awake and anaesthetized mice. Right: quantifications of glucose consumption based on 14 C-2DG autoradiography in the cortex of awake and ketamine/xylazine-anaesthetized mice. P =0.001, t -test ( N =5). ( b ) Left: imaging of 2DG-IR in the cortex of awake and mice anaesthetized with ketamine 100 mg kg −1 and xylazine 10 mg kg −1 , intraperitoneally (i.p. ; KX). Scale bars, 20 μm. Right: anaesthesia reduced the ratio of neuronal versus astrocytic 2DG-IR uptake in the cortex. P =0.002, Mann–Whitney test, N =9 awake, N =6, anaesthetized. Bar graphs represent mean±s.e.m. Full size image Sensory stimulation increases neuronal glucose uptake In a revised version of the lactate shuttle hypothesis, it is proposed that activity-induced increases in glucose uptake reflect astrocytic glucose uptake, and that astrocytes in turn produce lactate, which is oxidized by neurons [29] . To test this hypothesis, we first evaluated how functional neuronal activation affects local 2DG-IR uptake. The mice were fasted before the experiment, to reduce the potential effect of astrocytes’ glycogen stores on cerebral metabolism [30] , [31] , [32] , [33] . We stimulated the whiskers (3 Hz) unilaterally in awake mice and used local field potential (LFP) recordings to confirm that the whisker deflections induced neural responses in the contralateral barrel cortex for the duration of the stimulation period ( Fig. 5a ). We compared 2DG-IR uptake in ipsi- and contralateral sensory cortex and found that whisker stimulation significantly increased 2DG-IR uptake in contralateral compared with ipsilateral barrel cortex ( Figs 5b,d ). A microscopic analysis of 2DG-IR uptake showed that whisker stimulation predominantly increased 2DG-IR uptake in neurons, as the ratio of 2DG-IR signal in neurons versus astrocytes increased from 2.1-fold to 3.3-fold in contra- versus ipsilateral barrel cortex of awake mice ( P =0.006, t -test, Fig. 5e–g ). In fact, 2DG-IR signal intensity in astrocytes did not exhibit an increase in contralateral barrel cortex compared with ipsilateral (41.3±9.4 au in contralateral and 50.2±8.8 au in ipsilateral, P =0.51, t -test, N =7 contralateral and N =9 ipsilateral). Analysis of glucose metabolism based on traditional 14 C-2DG autoradiography showed, in accordance with previous analysis, a significant increase in glucose consumption in the contralateral barrel cortex (19±4%, P <0.01, t -test, Fig. 5c ) [34] . Thus, based on these observations, we conclude that sensory stimulation triggers an increase in glucose uptake preferentially by neurons. 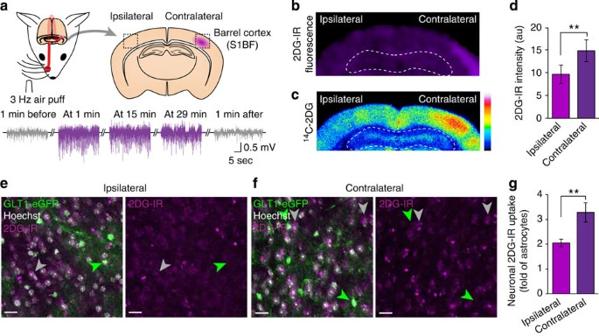Figure 5: Functional activation increases neuronal uptake, but not astrocytic uptake of 2DG-IR. (a) Upper panel: diagram of experimental setup. Whisker stimulation (air puffs, 3 Hz, 30 min) induced an increase in uptake of 2DG-IR and14C-2DG in contralateral somatosensory barrel cortex (S1BF). Lower panel: LFP recording in contralateral cortex 1 min before, 1, 15 and 29 min into the stimulation and 1 min after whisker stimulation. (b) Representative images of 2DG-IR fluorescence and (c)14C-2DG autoradiography of whisker stimulated mice. White dotted lines outline hippocampus. Contralateral cortex was 19±4% higher than ipsilateral cortex.P<0.01, pairedttest (N=5). (d) Quantification of 2DG-IR fluorescence in contralateral and ipsilateral barrel cortex in mice with whisker stimulation.P=0.003, pairedt-test (N=7). Representative images of 2DG-IR uptake in neurons and astrocytes in (e) ipsilateral and (f) contralateral cortex of whisker stimulated mice. Scale bars, 20 μm. Right panel: close-up images of 2DGIR in neurons and astrocytes in ipsi- and contralateral cortex with and without eGFP and yellow-Hoechst signals. (g) Quantification of 2DG-IR fluorescence in neurons relative to astrocytes in the respective regions.P=0.006,ttest (N=7 contralateral andN=9 ipsilateral). Bar graphs represent mean±s.e.m. Figure 5: Functional activation increases neuronal uptake, but not astrocytic uptake of 2DG-IR. ( a ) Upper panel: diagram of experimental setup. Whisker stimulation (air puffs, 3 Hz, 30 min) induced an increase in uptake of 2DG-IR and 14 C-2DG in contralateral somatosensory barrel cortex (S1BF). Lower panel: LFP recording in contralateral cortex 1 min before, 1, 15 and 29 min into the stimulation and 1 min after whisker stimulation. ( b ) Representative images of 2DG-IR fluorescence and ( c ) 14 C-2DG autoradiography of whisker stimulated mice. White dotted lines outline hippocampus. Contralateral cortex was 19±4% higher than ipsilateral cortex. P <0.01, paired t test ( N =5). ( d ) Quantification of 2DG-IR fluorescence in contralateral and ipsilateral barrel cortex in mice with whisker stimulation. P =0.003, paired t -test ( N =7). Representative images of 2DG-IR uptake in neurons and astrocytes in ( e ) ipsilateral and ( f ) contralateral cortex of whisker stimulated mice. Scale bars, 20 μm. Right panel: close-up images of 2DGIR in neurons and astrocytes in ipsi- and contralateral cortex with and without eGFP and yellow-Hoechst signals. ( g ) Quantification of 2DG-IR fluorescence in neurons relative to astrocytes in the respective regions. P =0.006, t test ( N =7 contralateral and N =9 ipsilateral). Bar graphs represent mean±s.e.m. Full size image HK expression is mainly neuronal and correlates with glucose consumption From the astrocyte-to-neuron lactate shuttle hypothesis, it follows that the level of glycolysis is required to be higher in astrocytes than neurons, and thus HKs should be expressed preferentially in astrocytes. Gene expression analysis of fluorescence-activated cell (FACS)-sorted pools of cortical neurons and astrocytes showed that both cell types express HK enzymes, as expected [33] , [35] , [36] . However, the quantitative PCR (qPCR) data of the messenger RNA revealed that the HK1 , HK2 and HK3 genes were consistently expressed at a higher level in neurons than in astrocytes ( Fig. 6a ) [37] . Using quantitative immunohistochemical analysis, we confirmed the gene expression data: HK1, HK2 and HK3 immunolabelling were significantly higher in neurons than in astrocytes ( Fig. 6b–k and Fig. 7a–e ). The higher expression of the HK1–3 in neurons compared with astrocytes was not limited to the cortex, but evident in all regions analysed, including the striatum and hippocampal layers CA1 and CA3 ( Figs 6b–k and 7a–e ). Vascular endfeet of astrocytes were easily recognized in the GLT1-eGFP reporter mice and displayed, similar to parenchymal astrocytes, low levels of HK ( Fig. 6c,d ). Thus, both qPCR and immunohistochemistry data suggested that the capacity for glucose phosphorylation, and therefore glycolysis, in neurons by far exceeds that of astrocytes. The observations that neurons take up more glucose and express several fold higher glycolytic enzymes (HK1–3) compared with astrocytes support the claim that neurons are the primary consumers of glucose ( Figs 6b–k and 7a–e ). Plotting local glucose consumption as a function of local HK1 expression across several brain regions confirmed a linear relationship ( R 2 =0.78, Fig. 8a,b ) [17] . Moreover, this observation was extended by the observation that the 2DG-IR uptake ratio for neurons versus astrocytes was also a function of local HK1 expression ( R 2 =0.85, Fig. 8c ). These data emphasize the notion that HK expression on a macroscopic level (comparing brain regions), as well as on a microscopic level (comparing different cell types) is a direct function of the basal level of glucose metabolism. Both the macro- and microscopic analysis of HK expression suggested that glucose is primarily used by neurons. Finally, we investigated the level of HK1, also called ‘brain HK’, in adult human cortex [38] . HK1 immunofluorescence signal was localized predominantly to NeuN + neurons, which consistently displayed stronger HK1 immunolabelling than Glial Acidic Fibrillary Protein (GFAP)-positive astrocytes ( Fig. 8d,e ), supporting the hypothesis that glycolysis is an integral constituent of neuronal ATP production in both murine and human brain. 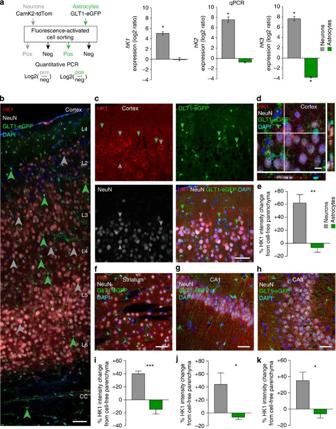Figure 6: Neurons express high levels of hexokinases. (a) Left: diagram of FACS sorting strategy for qPCR ofhK1-3. Right: qPCR analysis ofhK1–3expression in FACS-sorted cortical neurons (tdTomato+versus tdTomato−cell population harvested from Camk2a-CreERT2/CAG-tdTomato reporter mice) and astrocytes (eGFP+versus eGFP−cell populations harvested from GLT1-eGFP reporter mice) expressed as log2 of the ratio of positive versus negative population.P<0.05 compared with negative populations forhK1–3in neurons andhK3in astrocytes (N=3 mice in each group). (b,c) Immunohistochemistry of HK1 (red) in neurons (NeuN+, grey arrow) and astrocytes (green arrow, eGFP+) with DAPI (blue) in the cortex of a GLT1-eGFP reporter mouse. Scale bar, 50 μm. (d) Orthogonal projections of a 0.1-μm step size Z-stack. Green arrow indicates an astrocyte endfoot. (e) Quantification of HK1 immunoflourescence shown in percentage difference in HK1 immunolabelling intensity relative to cell-free parenchyma in the cytosol of NeuN+neurons (grey) and GLT1-eGFP+astrocytes (green) in the cortex.P<0.01,t-test (40 neurons and 40 astrocytes fromN=4 mice). (f–h) Immunohistochemistry of HK1 and NeuN in GLT1-eGFP mouse and (i–k) percentage difference in immunolabelling intensity relative to cell-free parenchyma in the striatum, CA1 and CA3, respectively. Scale bars, 50 μm (f–h);P<0.001 for the striatum,P<0.05 for CA1 and CA3,t-test (40 neurons and 40 astrocytes inN=4 mice). Bar graphs represent mean±s.e.m. Figure 6: Neurons express high levels of hexokinases. ( a ) Left: diagram of FACS sorting strategy for qPCR of hK1-3 . Right: qPCR analysis of hK1–3 expression in FACS-sorted cortical neurons (tdTomato + versus tdTomato − cell population harvested from Camk2a-CreERT2/CAG-tdTomato reporter mice) and astrocytes (eGFP + versus eGFP − cell populations harvested from GLT1-eGFP reporter mice) expressed as log2 of the ratio of positive versus negative population. P <0.05 compared with negative populations for hK1–3 in neurons and hK3 in astrocytes ( N =3 mice in each group). ( b , c ) Immunohistochemistry of HK1 (red) in neurons (NeuN + , grey arrow) and astrocytes (green arrow, eGFP + ) with DAPI (blue) in the cortex of a GLT1-eGFP reporter mouse. Scale bar, 50 μm. ( d ) Orthogonal projections of a 0.1-μm step size Z-stack. Green arrow indicates an astrocyte endfoot. ( e ) Quantification of HK1 immunoflourescence shown in percentage difference in HK1 immunolabelling intensity relative to cell-free parenchyma in the cytosol of NeuN + neurons (grey) and GLT1-eGFP + astrocytes (green) in the cortex. P <0.01, t -test (40 neurons and 40 astrocytes from N =4 mice). ( f – h ) Immunohistochemistry of HK1 and NeuN in GLT1-eGFP mouse and ( i – k ) percentage difference in immunolabelling intensity relative to cell-free parenchyma in the striatum, CA1 and CA3, respectively. Scale bars, 50 μm ( f – h ); P <0.001 for the striatum, P <0.05 for CA1 and CA3, t -test (40 neurons and 40 astrocytes in N =4 mice). Bar graphs represent mean±s.e.m. 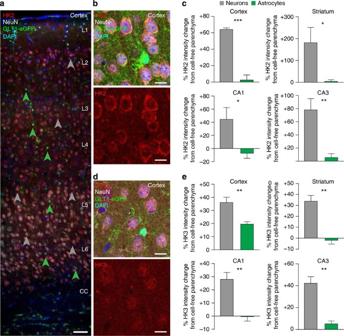Figure 7: Neurons express high levels of HK2 and 3. (a) Immunohistochemistry of HK2 (red) in neurons (NeuN+, grey arrow) and astrocytes (green arrow, eGFP+) with DAPI (blue) of a GLT1-eGFP reporter mouse from the surface of cortex through to the corpus callosum. Scale bar, 50 μm. (b) HK2 (red) and NeuN (white) immunohistochemistry in GLT1-eGFP mouse cortex. Scale bar, 50 μm. (c) Percentage difference in HK2 immunolabelling intensity relative to cell-free parenchyma in the cytosol of NeuN+neurons (grey) and GLT1-eGFP+astrocytes (green) in the cortex (P<0.001), striatum (P<0.05), CA1 (P<0.05) and CA3 (P<0.01),t-test (30–50 neurons and 30–50 astrocytes inN=4 mice). (d) HK3 (red) and NeuN (white) immunohistochemistry in GLT1-eGFP mouse cortex. Scale bar, 50 μm. (e) Percentage difference in HK3 immunolabelling intensity relative to cell-free parenchyma in the cytosol of NeuN+neurons (grey) and GLT1-eGFP+astrocytes (green) in the cortex, striatum, CA1 and CA3.P<0.01,t-test (35–50 neurons and 35–50 astrocytes inN=4 mice). Bar graphs represent mean±s.e.m. Full size image Figure 7: Neurons express high levels of HK2 and 3. ( a ) Immunohistochemistry of HK2 (red) in neurons (NeuN + , grey arrow) and astrocytes (green arrow, eGFP + ) with DAPI (blue) of a GLT1-eGFP reporter mouse from the surface of cortex through to the corpus callosum. Scale bar, 50 μm. ( b ) HK2 (red) and NeuN (white) immunohistochemistry in GLT1-eGFP mouse cortex. Scale bar, 50 μm. ( c ) Percentage difference in HK2 immunolabelling intensity relative to cell-free parenchyma in the cytosol of NeuN + neurons (grey) and GLT1-eGFP + astrocytes (green) in the cortex ( P <0.001), striatum ( P <0.05), CA1 ( P <0.05) and CA3 ( P <0.01), t -test (30–50 neurons and 30–50 astrocytes in N =4 mice). ( d ) HK3 (red) and NeuN (white) immunohistochemistry in GLT1-eGFP mouse cortex. Scale bar, 50 μm. ( e ) Percentage difference in HK3 immunolabelling intensity relative to cell-free parenchyma in the cytosol of NeuN + neurons (grey) and GLT1-eGFP + astrocytes (green) in the cortex, striatum, CA1 and CA3. P <0.01, t -test (35–50 neurons and 35–50 astrocytes in N =4 mice). Bar graphs represent mean±s.e.m. 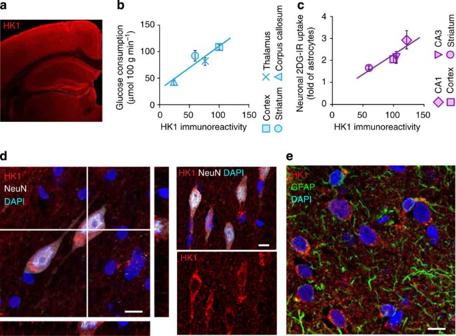Figure 8: Correlation of hexokinase with glucose consumption and its expression in human brain. (a) HK1 immunohistochemistry of mouse brain. (b) Glucose consumption calculated from14C-2DG signal in the cortex, striatum, thalamus, and corpus callosum plotted against HK1 immunoreactivity in the same area. Correlation coefficientR2=0.85 (N=5 for HK1 quantification,N=5 for autoradiography). (c) The ratio of neuronal versus astrocytic 2DG-IR uptake plotted against HK1 immunoreactivity in the cortex, striatum, hippocampal CA1 and CA3 regions. Correlation coefficientR2=0.78 (N=5 for HK1 quantification,N=6–9 for 2DG-IR uptake). (d) Orthogonal projections of a 0.1-μm step size Z-stack and image of HK1 (red) and NeuN (grey) immunohistochemistry of adult human cortex. (e) Immunohistochemistry of HK1 (red) and GFAP (green) in adult human cortex. Scale bars, 10 μm (d,e). Full size image Figure 8: Correlation of hexokinase with glucose consumption and its expression in human brain. ( a ) HK1 immunohistochemistry of mouse brain. ( b ) Glucose consumption calculated from 14 C-2DG signal in the cortex, striatum, thalamus, and corpus callosum plotted against HK1 immunoreactivity in the same area. Correlation coefficient R 2 =0.85 ( N =5 for HK1 quantification, N =5 for autoradiography). ( c ) The ratio of neuronal versus astrocytic 2DG-IR uptake plotted against HK1 immunoreactivity in the cortex, striatum, hippocampal CA1 and CA3 regions. Correlation coefficient R 2 =0.78 ( N =5 for HK1 quantification, N =6–9 for 2DG-IR uptake). ( d ) Orthogonal projections of a 0.1-μm step size Z-stack and image of HK1 (red) and NeuN (grey) immunohistochemistry of adult human cortex. ( e ) Immunohistochemistry of HK1 (red) and GFAP (green) in adult human cortex. Scale bars, 10 μm ( d , e ). Full size image In this study, we analysed neuronal and astrocytic uptake of a near-infrared glucose analogue, 2DG-IR in vivo using two-photon microscopy. Initial in vitro analysis validated that uptake of 2DG-IR follows similar uptake and inhibition kinetics as glucose and 2DG in both cultured neurons and astrocytes. The in vitro analysis also documented that neuronal uptake of glucose itself is fourfold higher than astrocytes in cultures. In vivo , we delivered 2DG-IR directly into CSF of awake behaving reporter mice to visualize cellular 2DG-IR uptake. Real-time imaging showed that 2DG-IR entered cortex along penetrating arteries and reached the capillary bed by convective transport along the perivascular space, followed by uptake by both neurons and astrocytes. Quantitative analysis of cellular 2DG-IR uptake indicated that the glucose analogue was preferentially taken up by neurons in awake animals, and that ketamine/xylazine anaesthesia predominantly suppressed neuronal glucose metabolism. In addition, whisker stimulation increased neuronal, rather than astrocytic, 2DG-IR uptake in awake mice. Thus, our analysis showed that neurons consistently take up more glucose than astrocytes across several fundamentally different states of brain activity. Another important conclusion is that glucose metabolism should be studied in awake rather than anaesthetized animals, as anaesthesia preferentially suppresses neuronal 2DG-IR uptake. HKs are housekeeping enzymes that catalyse the first step of glycolysis [35] , [36] . Analysis of gene expression in FACS-sorted neuron and astrocytes showed that all three isoforms of HK ( hK1–3 ) are expressed at higher levels in neurons than in astrocytes. A quantitative immunohistochemical analysis confirmed and extended this observation by showing that HK1–3 are present at higher levels in neurons than in astrocytes in all brain regions analysed. The enrichment of HK1 in NeuN-positive neurons is in agreement with the observation that 40%–50% of HK activity is localized in synaptosomes [39] . We also confirmed that regional HK1 expression correlates with local glucose utilization [17] , and extended this observation to demonstrate that the ratio of neuron/astrocyte glucose uptake correlates with HK1 content in the same regions. In human cortex, an assessment of the prevailing hexokinase, HK1 (refs 38 , 40 ) revealed a much stronger HK1 immunolabelling of NeuN + neurons than GFAP + astrocytes, suggesting that our observations in mice can be extended to the human brain. An additional important observation was that HK1 was not enriched in vascular endfeet of astrocytes, as would be expected according to the astrocyte-to-neuron lactate shuttle hypothesis. In combination, our observations are consistent with the simple model that neurons, rather than astrocytes, are the primary direct consumers of glucose. The CNS consumes tenfold more energy than the average of peripheral tissue and relies almost exclusively on glucose as energy substrate [20] , [41] , [42] . According to the astrocyte–to-neuron lactate shuttle hypothesis, glucose uptake is delegated to astrocytes and neurons rely chiefly on import of lactate from nearby astrocytes. The concept of the astrocyte-to-neuron lactate shuttle was originally based on the observation that glutamate uptake in cultured astrocytes activated aerobic glycolysis, leading to an increased astrocytic production of lactate [8] . Accordingly, glutamatergic signalling enhances astrocytic lactate production and lactate is in turn imported and oxidized by neurons. Several experiments have in the past supported the existence of astrocyte-to-neuron lactate shuttle hypothesis [4] , [6] , [8] , [29] . In vitro studies have used shorter wavelength glucose analogues, including 2-NBDG and 6-NBDG, to compare the uptake kinetics in cultured neurons and astrocytes [22] . However, comparison of transport kinetics in different cell types is complicated, because the glucose transporter isoforms differ with regard to affinity and transport kinetics [19] . Neurons express primarily GLUT3, whereas GLUT1 is highly enriched in astrocytes [18] , [19] . One prior study assessed 2-NBDG accumulation in vitro , rather than its transport kinetics, and concluded that the glucose analogue is primarily taken up by neurons, consistent with our findings [43] , [44] . Data collected in brain slices incubated with fluorescent glucose analogues have also supported the astrocyte-to-neuron lactate shuttle hypothesis [45] , [46] . However, interpretation of the slice data is difficult, as glucose is not delivered by the vasculature and astrocytes rapidly acquire a reactive phenotype ex vivo [47] . An analysis based on in vivo imaging of the glucose analogue, 6NBDG, at rest and during functional activation in anaesthetized mice concluded, as opposed to our study, that neurons take up more glucose than astrocytes [48] . However, C6-conjugated glucose analogues cannot be phosphorylated by the HKs (which target the C6 site occupied by the fluorescent tag), in contrast to the classical glucose analogues used in quantitative assessment of glucose consumption, including the 2DG derivative, 18 FDG, 2NBDG, or 2DG-IR. Consequently, 6NBDG is not trapped within the cells rendering it is difficult to compare neuronal versus astrocytic uptake [26] , [49] . Definitive proofs for or against the existence of the astrocyte-to-neuron lactate shuttle in vivo have also been hampered by the lack of cellular resolution of the classical autoradiographic analysis of radiolabelled 2DG [50] . Two prior studies attempted to overcome this limitation by applying emulsion directly on the sections. Albeit the majority of the grains were located over large cell bodies, consistent with the high HK expression in neuronal cell bodies, the lack of immunolabelling prevented definitive cell identification [12] , [51] . The glucose analogue used in this study, 2DG-IR, was developed for infrared non-invasive imaging of tumours with high glucose consumption [13] , [14] . Long wavelength excitation and emission have several advantages, including better tissue penetration, less scattering and low autofluorescence. 2DG-IR has, to our knowledge, not previously been employed in analysis of cerebral metabolism. We took advantage of the fact that small tracers are rapidly distributed brain-wide by convective fluxes of CSF and bypassed thereby the poor permeability of fluorescently tagged glucose analogues across the BBB [25] . Our analysis confirmed that 2DG-IR, within minutes, was transported along the peri-arterial and peri-capillary space, and shortly thereafter distributed evenly across all brain regions. In fact, delivery of glucose analogues by convective CSF influx via the glymphatic system closely replicates vascular delivery of glucose, because both pathways require that the glucose tracers crosses the peri-capillary space before gaining access to either astrocytes and neurons ( Fig. 1a ). The even distribution of 2DG-IR across all brain regions suggests that cisterna magna injection of agents with poor BBB permeability may also be a useful tool for other studies that require brain-wide distribution including pharmacological manipulations, loading of fluorescent indicators or viral transfection. We perfusion-fixed the mice 30 min after in vivo 2DG-IR administration and prepared vibratome sections immediately thereafter. The 2DG-IR signal in intact cells was collected using 1,280 nm excitation in the slices. The intactness of the plasma membrane following perfusion–fixation was, in pilot experiments, evaluated by imaging the same field repeated over a period of 24 h. This analysis showed that the cellular signals did not change significantly over time, suggesting that the intact plasma membrane prevented diffusion of the glucose analogue trapped within the plasma membrane. This observation is in agreement with earlier studies, in which fine cellular structures were visualized by intracellular injection of fluorescent indicators in freshly cut slices of perfusion-fixed animals [52] . We also used transgenic reporter mice (GLT1-eGFP) to positively label astrocytes and yellow Hoechst, to identify surrounding neurons based on the large size of neuronal nuclei, as well as loose chromatin structure with multiple nucleoli and lack of eGFP. In combination, these technical advances improved the cellular details of the 2DG-IR signal and allowed with high specificity quantification of glucose uptake in neurons and astrocytes located next to each other across multiple brain regions and three different states of brain activity. Our analysis confirms a recent study in anaesthetized rats, which showed that bicuculline-induced seizures increased 18 F-DG phosphorylation in isolated nerve terminals, suggesting that local neuronal glycolysis supports increased synaptic activity [11] . The activity of HKs is inhibited by ATP and the product of their own reaction, glucose-6-phosphate, and it has been estimated that HK activity is 97% inhibited at rest [53] . Thus, a decline in cytosolic ATP and glucose-6-phosphate in rapidly spiking neurons may drive neuronal, rather than astrocytic, glucose consumption during functional activation. This conclusion is of importance, because metabolic surrogates of metabolism are widely employed in functional imaging studies [54] , [55] , [56] , [57] . However, interpretation of functional autoradiographic and PET studies based on radiolabelled ( 14 C or 3 H) 2DG and 18 FDG, respectively, have been complicated by the astrocyte-to-neuron lactate shuttle hypothesis. The data presented here provide insight into the cellular basis for functional brain imaging, by showing that glucose is taken up by neurons in an activity-dependent manner, and that regional 2DG or 18 FDG accumulation thereby can be used as direct measure of neuronal activity. In future experiments, imaging glucose uptake based on administration of 2DG-IR in the CSF provides a new experimental approach to dissect cellular metabolic responses to state-dependent changes in neural activity or pathological conditions such as ischaemia, epilepsy or neurodegenerative diseases. Mice All mice were 2–3 months old ( ∼ 25 g) unless otherwise stated. Camk2a-CreERT2/CAG-tdTomato (Camk2a-tdTomato) mice were generated by crossing B6.129S6-Tg (Camk2a-cre/ERT2)1Aibs/J mice and B6.Cg- Gt(ROSA)26Sor tm14(CAG-tdTomato)Hze /J (Jackson) [58] , [59] , [60] . At 5 weeks of age, tamoxifen (Sigma; T5648) was injected (150 mg kg −1 , intraperitoneally) daily for 7 consecutive days. BAC GLT1-eGFP (GLT1-eGFP) [61] mice were used as astrocyte reporter mice. All strains were maintained on C57BL/6J background and C57BL/6NCrl mice were purchased from Charles River Laboratory to rejuvenate the transgenic lines. All experiments were approved by the University Committee on Animal Resources of the University of Rochester and carried out according to guidelines from the National Institute of Health. FACS analysis and RNA extraction Eight-week-old Camk2a-tdTomato and GLT1-eGFP mice were used for isolating neurons and astrocytes, respectively. Preparation of single cell suspension from mouse cortex and hippocampus, and FACS analysis were performed as described previously [37] , [62] . Cortical tissue from three mice was pooled for one sample, with a yield of 4 ∼ 8 × 10 6 cells per mouse. A 561- and 488-nm laser was used for tdTomato and eGFP excitation, respectively, and emissions were collected by a 610/20- and 530/30-nm band-pass filter, respectively. Cells were sorted into either tdTomato + (neurons) and tdTomato − , or eGFP + (astrocytes) and eGFP − populations. RNA of FACS-sorted cells was extracted using RNeasy Micro Kit (Qiagen) [37] . Quantitative PCR For qPCR, total RNA was reverse transcribed and amplified using Ovation PicoSL WTA System V2 (NuGEN). Relative quantity of transcripts was assessed using Taqman Assays on Demand and a 7000 Sequence Detection System. Expression of synaptosomal-associated protein 25 (Snap25) and embryonic lethal abnormal vision drosophila-like 4 in neurons, solute carrier family 1, member 2 and aquaporin 4 in astrocytes, and the absence of integrin, alpha M (microglia) and myelin oligodendrocyte glycoprotein (oligodendrocytes) expression were used to verify sorting specificity. RNA quantity was normalized to glyceraldehyde 3-phosphate dehydrogenase before calculating relative expression of target genes [63] . Values were expressed as log2 of the ratio of the relative expression ratio of target gene in Camk2a + /Camk2a − or GLT1 + /GLT1 − cells. Cell cultures Neocortical astrocyte cultures were prepared from 1- to 2-day-old GLT1-eGFP mice [64] . Astrocytes were plated in 25 cm 2 culture flask (10 6 cells per flask) and maintained in 10% fetal bovine serum in DMEM/F12, containing penicillin (100 IU ml −1 ) and streptomycin (100 μg ml −1 ). When the cultures became confluent, the cells were re-plated in 24-well plates (2 × 10 5 cells per well). Experiments were performed when the cells were 90% confluent, about 2 days after seeding down. Neocortical neuronal cultures were prepared from 1 - to 5-day-old C57BL/6 mice as previously described [64] . The cells were seeded onto poly- D -lysine-coated 24-well plates (10 5 cells per well) and maintained in Neurobasal A medium (Invitrogen) with 2% B27, 0.5 mM GlutaMAX, gentamycin (10 μg ml −1 ) and human fibroblast growth factor 2 (5 ng ml −1 ). Neuronal cultures were used 7 days after plating. More than 95% of the cells stained positive for GFAP in the astrocyte cultures and >95% of the cells stained positive for PSA-NCAM in the neuronal cultures (see Methods section for immunohistochemistry and image analysis). Cell culture assays Neuron and astrocyte cultures, 90% confluent, in 24-well plates were washed twice and pre-incubated in 0.5 mM D -glucose (Sigma) in DMEM for 30 min at 37 °C (refs 64 , 65 ). The assay media contained 0.5 mM D -glucose and D [U- 14 C]-glucose ( 14 C-glucose), or glucose analogues 2[ 14 C(U)-deoxy- D -glucose ( 14 C-2DG) or IRDye 800CW-2-deoxyglucose (2DG-IR, LI-COR Biosciences, Nebraska, USA) in DMEM [8] , [66] . All experiments were performed at 37 °C. At the end of the experiment, the cells were washed three times with 0.5 ml ice-cold glucose-free DMEM containing 0.5 mM glucose. For 14 C-glucose and 14 C-2DG experiments, 1 μCi ml −1 (0.5 mM, PerkinElmer, MA, USA) was used and at the end of the experiment the cells were lysed in 200 μl 0.5 N NaOH/0.1% Triton X-100. Protein concentration was determined by Pierce BCA protein assay kit (Thermo Scientific). 14 C radioactivity was quantified using a liquid scintillation counter (LS6500 Scintillation Counter, Beckman Coulter, GA, USA). For 2DG-IR uptake experiments, assays were performed in 96-well plates with 100 μM 2DG-IR in the assay media. After incubation with 2DG-IR, followed by three quick washes, 2DG-IR signal was imaged in three random places per well using a 20 × water immersion lens (0.95 numerical aperture (NA)). Mean pixel intensity was measured using NIH ImageJ 1.47v software and background intensity measurement (blank well with media) was subtracted. Assay times for 14 C-glucose, 14 C-2DG and 2DG-IR were 1, 2, 6 or 10 min. The initial rate of uptake was determined by linear regression analysis from the initial linear phase of the uptake versus time graph. Uptake inhibition experiments with addition of D -glucose (in mM: 0, 0.1, 0.2, 0.3, 1, 3, 10, 30, 100 and 300; Sigma) or cytochalasin B (in μM: 0, 1, 5, 10, 20 and 40; Sigma) to the assay media, DMEM containing 0.5 mM D -glucose, were performed at 1 min. For 2DG-IR competition and inhibition experiments, 10 μM 2DG-IR was added to the assay media and the well plate was imaged using an IVIS spectrum imaging system (Caliper Life Science, MA, USA), and the mean fluorescence signal was used. Uptake of 14 C-glucose and 4 C-2DG was expressed as nmol per mg protein, 2DG-IR was expressed as the mean fluorescence intensity. The inhibitory constant, K i , was calculated using Graph Pad Prism 5. All experiments were performed in triplicate. Immunohistochemistry and image analysis Immunohistochemistry was performed as previously described [67] . The primary antibodies used were: mouse anti-HK1 (1:250, Millipore MAB1534), rabbit anti-HK2 (Millipore AB3279, 1:200), rabbit anti-HK3 (Santa Cruz sc-28890, 1:100), mouse anti-NeuN (Chemicon MAB377, 1:200), rabbit anti-NeuN (Millipore ABN78, 1:250), rabbit anti-GFAP (DAKO Z0334, 1:250) and mouse anti-PSA-NCAM (Millipore MAB5324, 1:250). Alexa Fluor-conjugated secondary antibodies were incubated for 2 h at room temperature (Life Technologies, 1:500). DAPI (4,6-diamidino-2-phenylindole; Sigma, 1:2,000) was used to identify cell nuclei. For immunohistochemistry on human tissue, the tissue was immersion fixed in 4% paraformaldehyde, embedded in O.C.T. Tissue-Tek (Sakura) and cut in 20 μm cryostat sections. A biotinylated secondary antibody (1:200) directed against HK1 primary antibody was used. Alexa Fluor-conjugated streptavidin (20 μg /ml −1 ) was applied for 2 h. Immunofluorescence was visualized using a Bio-Rad MRC500 confocal scanning microscope attached to an inverted microscope (IX81, Olympus, Tokyo, Japan) controlled by Olympus Fluoview 500 software. A × 4 lens (0.16 NA) was used to image HK immunofluorescence for comparison of different brain regions, a × 10 lens (0.3 NA) was used for imaging of immunocytochemistry, a × 40 lens (1.3 NA) was used for imaging of immunocytochemistry for cellular HK quantification and a × 100 lens (1.3 NA) was used for Z-stacks. A Z-stack of 0.1 μm steps was acquired for orthogonal projections ( xz , yz plane). Orthogonal projections were made using Olympus Fluoview 500 software [47] . For analysis of HK protein, immunohistochemistry was performed on 100 μm vibratome slices of GLT1-eGFP mice. Neurons were identified by NeuN labelling. Astrocytes were identified by eGFP expression. NIH ImageJ software 1.47v was used to measure HK1 immunoreacticity intensity. The intensity of HK1 immunoreactivity in the nucleus (co-localization with DAPI) was subtracted from the HK1 intensity in the soma, to yield the cytoplasmic HK1 immunoreactivity intensity. Background intensities (>3 per image) were measured in cell-free parenchyma in the same field of view and the data were displayed as the percentage difference between neuronal and astrocytic fluorescence intensity, respetively, compared with cell-free parenchyma. Cell-free parenchyma was defined as space devoid of eGFP, NeuN or DAPI, but could contain some unidentified cellular processes of, for example, astrocytes or neurons. A total of 30–50 neurons and 30–50 astrocytes per brain region were quantified in N =4 mice. For comparison of HK immunoreactivity in different brain regions, images were normalized to the intensity measure in the cortex of each sample ( N =5). Awake whisker stimulation and electrophysiological recording Adult GLT1-eGFP mice underwent adaptive behavioural training for awake restraining using several 1 h sessions over two consecutive days. The mice were fasted overnight before the day of the experiment. Whiskers were trimmed to 10-mm length and stimulated by air puffs [68] . The tube for air puffing was placed parallel to the left side of the mouse snout 15–20 mm in front of the C6 whisker. Air puffs controlled by a picospritzer (Parker Instrumentation) were generated at 3 Hz, 20 psi, 10 ms pulses for a duration of 30 min. LFP recordings were obtained from primary sensory cortex (100–150 μm below the pial surface) by a patch pipette (TW100F-4, WPI; outer diameter, 1.0 mm; inner diameter, 0.75 mm; tip diameter, 3 μm), containing artificial CSF (in mM): 126 NaCl, 2.5 KCl, 1.25 NaH 2 PO 4 , 2 MgCl 2 , 2 CaCl 2 , 10 glucose and 26 NaHCO 3 (pH 7.4). LFP signals were amplified by a MultiClamp 700B (Axon Instruments), bandpass filtered at (1–100 Hz) and digitized at 10 kHz [68] . Animal preparation for in vivo two-photon imaging GLT1-eGFP mice and Camk2a-tdTomato mice were anaesthetized with 2% isoflurane in 2 l O 2 per minute and a custom-made metal plate was glued to the skull with dental acrylic cement. The mice were habituated to the microscope stage over the following 2 days by several training session, each lasting 30–60 min. At day 2, the mice were fasted overnight. At day 3, the mice were anaesthetized with 2% isoflurane and a cranial window was prepared over the right hemisphere at 2.5 mm lateral and 2 mm posterior to bregma. The dura was left intact and the craniotomy ( ∼ 3 mm diameter) was covered with 1.5% agarose (type III-A, Sigma) and a glass coverslip, and then sealed with dental cement. All mice were allowed to recover for 4–6 h before imaging. In awake mice and mice anaesthetized with ketamine/xylazine (KX, 100 and 10 mg kg −1 , intraperitoneally) 2DG-IR was micro-injected along a penetrating arteriole in the cortex at a concentration of 1 mM using a fine glass electrode connected to a picospritzer (1 Hz, 10 psi, 100 ms pulses, for 10 min; Parker Instrumentation). To visualize the vasculature, the BBB impermeable Texas Red-dextran (70 kD, 1% in saline) or FITC-dextran (2,000 KDa, 1% in saline) was injected into the femoral vein of GLT1-eGFP mice and CamkIIa-tdTomato mice, respectively. Quantification of cellular 2DG-IR uptake in vivo Adult (>2 months old) GLT1-eGFP mice were used for 2DG-IR experiments. In one group, the mice were anaesthetized with KX, in another group the mice were awake. All awake mice received behavioural training described in the whisker stimulation section and all mice were fasted overnight before the experiment. The mice were infused with 20 μl of 1 mM 2DG-IR into cisterna magna (2 μl min −1 ). Whisker stimulation was initiated simultaneously with the start of 2DG-IR injection. The mice were perfused with 4% paraformaldehyde after 30 min. For comparison of 2DG-IR uptake by neurons and astrocytes, the brains were immediately sectioned in 100-μm-thick slices using vibratome, incubated with 40 μM yellow Hoechst in PBS (Life Technologies; S769121) for 20 min, washed twice in PBS for 10 min and mounted on a glass slide in Prolong (Invitrogen). All images were acquired using two-photon imaging with the same photomultiplier tube setting and gain for 2DG-IR within 2–3 h after perfusion fixation. Astrocytes were identified by cytosolic eGFP signal. Neurons were identified by their lack of eGFP and as cells with a round, lightly stained nuclei of >9 μm in size ( Fig. 3b ). A quantitative analysis showed that NeuN + nuclei were on average 43.7% larger in diameter than nuclei of GLT1-eGFP + astrocytes (10.2±0.7 μm for neurons, 7.1±0.1 μm for astrocytes, P =0.01, t -test, 82 neurons and 26 astrocytes quantified in N =3 mice). Measurements of 2DG-IR intensity were performed using NIH ImageJ 1.47v software. 2DG-IR background signal (measured in parenchyma) in the same field was subtracted from intensity measures in neurons and astrocytes in each image. In the cortex, the total number of neurons and astrocytes analysed were 333 and 125 for KX, 431 and 164 for awake/ipsilateral, and 387 and 140 for contralateral cortex, respectively. For analyses of other areas, 162±22 neurons and 59±4 astrocytes were analysed per mouse in N =7–8 mice. For imaging of 2DG-IR uptake in whole slices, an IVIS spectrum imaging system (Caliper Life Science) was used with an excitation and emission wavelength of 745 and 795 nm, respectively. A set of 20 images of whole-brain section was collected for each section and merged to generate a higher resolution final image. 2DG-IR content in the ipsilateral and contralateral barrel cortex and thalamus were quantified using NIH ImageJ software 1.47v. Two-photon imaging A Chameleon Ti:Sapphire laser (Coherent, Glasgow, UK) connected to a Chameleon compact opo system was controlled by Olympus Fluoview FV500 software [25] . A × 20 water immersion lens (0.95 NA) was used for in vivo and slice imaging. eGFP, 2,000 kDa dextran-FITC, 70 KDa dextran-Texas Red and yellow Hoechst were excited using a 900-nm laser. An 800 nm laser was tuned to 1,280 nm by the opo system for 2DG-IR excitation. Bandpass filters (Chroma) were 540/40 for eGFP and FITC, 650/75 nm for yellow Hoechst, 675/65 nm for tdTomato and Texas Red, and 855/210 nm for 2DG-IR emission. Single channel acquisition was used for 2DG-IR and dual channel acquisition was used for combination of other fluorophores. 14 C autoradiography Awake or KX-anaesthetized adult male C57BL/6 mice (25 g) were injected with 14 C-2DG (5 μCi/mouse, bolus) into the femoral vein. All mice were fasted overnight before the day of the experiment. Arterial blood samples (20 μl per sample) were collected before the injection for glucose determination and after the injection (11 samples during the experiment) for plasma radioactivity analysis. Total plasma glucose was determined using a kit (GAHK-20, Sigma). At the end of the experiments, mice were decapitated and their brains were embedded in O.C.T. Tissue-Tek (Sakura). Coronal sections (20 μm) were cut using a cryostat, collected on specimen glass slides, dried and exposed to autoradiographic film (Amersham Hyperfilm, GE Healthcare, UK) for 12 days with a 14 C- standard (American Radiolabeled Chemicals Inc., MO, USA). Intensity measurements of the developed films were performed using NIH ImageJ software 1.47v. Glucose utilization (μmol per 100 g min −1 ) was determined as: (Cp/LC) [C*(T)− k 1 * A ]/[ B − A ], where Cp is the plasma glucose concentration in mM, LC is the lump constant, C*(T) is 14 C-2DG in the brain region at time T , k 1 *, k 2 * and k 3 * are the influx, efflux and phosphorylation rate constants of 14 C-2DG, respectively, A = e −KT ∫ 0 T C* p ( t ) e Kt dt, B =∫ 0 T C p *( t )dt, K = k 2 *− k 3 * [26] , [27] , [28] , [49] , [69] . Statistics Values were expressed as mean±s.e.m. An unpaired Student’s t -test was used for pairwise comparisons. A paired t -test was used for analysis of neuronal 2DG-IR uptake normalized to astrocytic uptake in the same area. A Mann–Whitney test was used for pairwise comparison of data that did not follow normal distribution. Analysis of variance with Tukey–Kramer post-hoc test was used for comparisons of more than two groups. All statistics were performed using GraphPad Prism 5. How to cite this article: Lundgaard, I. et al . Direct neuronal glucose uptake heralds activity-dependent increases in cerebral metabolism. Nat. Commun. 6:7807 doi: 10.1038/ncomms7807 (2015).